Highly mesoporous metal–organic framework assembled in a switchable solvent The mesoporous metal–organic frameworks are a family of materials that have pore sizes ranging from 2 to 50 nm, which have shown promising applications in catalysis, adsorption, chemical sensing and so on. The preparation of mesoporous metal–organic frameworks usually needs the supramolecular or cooperative template strategy. Here we report the template-free assembly of mesoporous metal–organic frameworks by using CO 2 -expanded liquids as switchable solvents. The mesocellular metal–organic frameworks with large mesopores (13–23 nm) are formed, and their porosity properties can be easily adjusted by controlling CO 2 pressure. Moreover, the use of CO 2 can accelerate the reaction for metal–organic framework formation from metal salt and organic linker due to the viscosity-lowering effect of CO 2 , and the product can be recovered through CO 2 extraction. The as-synthesized mesocellular metal–organic frameworks are highly active in catalysing the aerobic oxidation of benzylic alcohols under mild temperature at atmospheric pressure. In recent years, metal–organic frameworks (MOFs) have attracted considerable attention because of their diverse fascinating topologies, pore size tenability and extensive uses in lots of fields such as catalysis, adsorption, chemical sensing and so on [1] , [2] , [3] . The construction of hierarchically meso- and microporous MOFs are of great interest, because they provide many novel properties and have important prospects in practical industrial processes [4] , [5] . The larger mesopores allow for improved molecular accessibility, whereas smaller micropores provide high surface areas. Some methods have been developed for the formation of hierarchically meso- and microporous MOFs, including surfactant–template method [6] , [7] , [8] , [9] , ligand extension method [10] , [11] , [12] , [13] , [14] , microwave-assisted method [15] , solvent evaporation diffusion method [16] , [17] , ionic liquid/supercritical CO 2 emulsion route [18] and so on. However, most of the meso-MOFs adopt smaller mesopores (<5 nm) and the preparation of large-pore meso-MOFs is sporadic at best, which usually needs the supramolecular or cooperative template strategy [6] , [9] . The augmentation of the MOF mesopores remains to be a major challenge. Compressed CO 2 has received much interest because it is nontoxic, inexpensive, non-flammable, and can be easily recaptured and recycled after use [19] , [20] , [21] . In particular, compressed CO 2 is quite soluble in many liquids, and can change the properties of the liquids considerably. For example, as CO 2 dissolves into an organic solvent, the liquid expands volumetrically, forming a CO 2 -expanded liquid (CXL) [22] . Therefore, by varying CO 2 pressure, a continuum of liquid media ranging from the neat organic solvent to CXL is generated, and their properties can be adjusted by tuning the operating pressure. Until now, CXLs have been shown to be optimal solvents in a variety of fields, including facilitating polymer processing [23] , [24] , [25] , [26] , serving as reaction media [27] , [28] , [29] , [30] , [31] , precipitating fine particles [32] , [33] , [34] , inducing separations [35] , [36] and so on. Herein, we propose the CO 2 -directed assembly of meso-MOFs. By using CXLs as switchable solvents, the mesocellular MOFs with large mesopores (13–23 nm) and ultra-high mesoporosities are formed. In comparison with the conventional methods for the meso-MOF formation, this strategy has many special advantages. First, the porosity properties of the as-synthesized MOFs can be easily modulated by CO 2 pressure. Second, the reaction for MOF formation from metal salt and organic linker can be accelerated by CO 2 due to the viscosity-lowering effect of CO 2 . Third, the product can be recovered through extracting the solvent by CO 2 . Fourth, CO 2 can be easily removed by reducing pressure. In addition, this method for the meso-MOF formation is template-free, involves no longer ligand, proceeds at room temperature and can be applied to the synthesis of different kinds of MOFs. The mesocellular MOFs have shown to be highly effective and reusable heterogeneous catalysts for aerobic oxidation of benzylic alcohols under mild temperature at atmospheric pressure. Volume expansion of the reaction system by CO 2 Cu 3 (BTC) 2 (H 2 O) 3 · x H 2 O (BTC=1,3,5-benzenetricarboxylate) is one of the most extensively explored MOFs for its various uses [6] , [9] , [37] , [38] , [39] . Herein we synthesized Cu 3 (BTC) 2 in CO 2 -expanded N , N -dimethylformamide (DMF) at 30 °C, using copper(II) acetate monohydrate (Cu(OAc) 2 ·H 2 O) and benzene-1,3,5-tricarboxylic acid (H 3 BTC) as MOF precursors. A certain amount of triethylamine was added into the reaction system to deprotonate the linker. 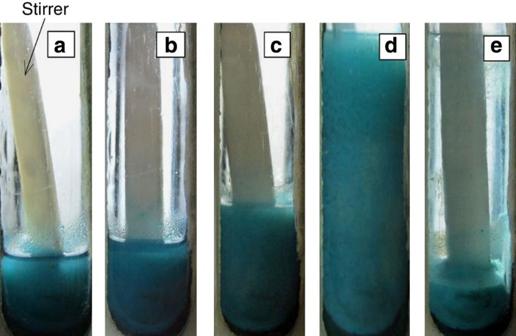Figure 1: Photographs of MOF synthesis in CO2-expanded DMF. (a) In pure DMF; (b) 2.0; (c) 4.5; (d) 6.6 MPa. (e) Phase separation in reaction system at 6.6 MPa after reaction for 3 h. Figure 1 shows the photographs of the reaction systems in pure DMF ( Fig. 1a ) and CO 2 -expanded DMF at different pressures ( Fig. 1b–d ). Evidently, the reaction system was expanded with the addition of CO 2 and the volume expansion increased at higher pressure. After 3 h of reaction the stirring was stopped. The product separated out from the solvent naturally and precipitated at the bottom of the autoclave ( Fig. 1e ). Then the upper solvent was extracted by flowing CO 2 , and the product precipitated at the bottom of the autoclave was recovered and washed using ethanol. Figure 1: Photographs of MOF synthesis in CO 2 -expanded DMF. ( a ) In pure DMF; ( b ) 2.0; ( c ) 4.5; ( d ) 6.6 MPa. ( e ) Phase separation in reaction system at 6.6 MPa after reaction for 3 h. Full size image Mesoporous Cu 3 (BTC) 2 synthesized in CO 2 -expanded DMF The Cu 3 (BTC) 2 synthesized in pure DMF (in the absence of CO 2 ) appeared as irregular agglomerates ( Supplementary Fig. 1 ). However, the mesocellular MOFs were formed in the CO 2 -expanded DMF. The Cu 3 (BTC) 2 synthesized at 2.0 MPa exhibits thick pore walls and mesopores of average size of 10 nm ( Fig. 2a,b ). When the pressure is increased to 4.5 MPa, the MOF is more porous, with thinner mesopore walls ( Fig. 2c,d ). The Cu 3 (BTC) 2 synthesized at 6.6 MPa has mesopores in 20–30 nm and the diameters of the pore walls are around 10 nm ( Fig. 2e,f ). Clearly, higher CO 2 pressure is favourable to form more porous MOFs, with larger mesopores and thinner pore walls. The X-ray diffraction (XRD) peak positions and relative intensities of the as-synthesized MOFs agree well with those of the simulated HKUST-1 (ref. 37 ; Supplementary Fig. 2 ). Fourier transform infrared spectra ( Supplementary Fig. 3 ) revealed that the carboxylate groups of H 3 BTC were coordinated to Cu(II) ions [9] , [18] , [40] . The characteristic C=O stretching vibration for acetic acid (1,770–1,750 cm −1 ) and C–N stretching vibration (1,230–1,030 cm −1 ) for triethylamine were not observed, indicating that the product is free of acetic acid and triethylamine, which could be removed easily by washing with ethanol. Energy-dispersive X-ray spectrum ( Supplementary Fig. 4 ) demonstrates the presence of copper, oxygen and carbon in the prepared MOF and no N element was detected, further proving the absence of triethylamine in the product. The MOFs could keep stable up to 310 °C, as evidenced by thermogravimetric analysis ( Supplementary Fig. 5 ), comparable to that of bulk HKUST-1 (refs 41 , 42 ). 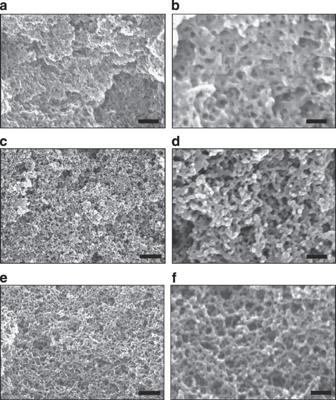Figure 2: SEM images of the Cu3(BTC)2synthesized in CO2-expanded DMF. (a,b) 2.0; (c,d) 4.5; (e,f) 6.6 MPa. Scale bars, 150, 50, 500, 150, 500 and 150 nm for (a–f), respectively. Figure 2: SEM images of the Cu 3 (BTC) 2 synthesized in CO 2 -expanded DMF. ( a , b ) 2.0; ( c , d ) 4.5; ( e , f ) 6.6 MPa. Scale bars, 150, 50, 500, 150, 500 and 150 nm for ( a – f ), respectively. Full size image Porosity properties of Cu 3 (BTC) 2 The porosity properties of the Cu 3 (BTC) 2 were determined by N 2 adsorption–desorption method after the sample was dried and degassed at 100 °C. 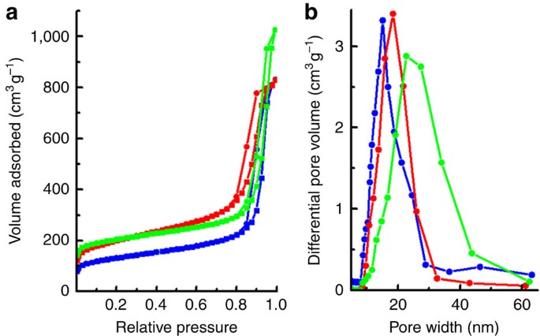Figure 3: Porosity measurements. Porosity properties of Cu3(BTC)2determined by N2adsorption–desorption method. (a) N2adsorption–desorption isotherms of the Cu3(BTC)2synthesized in CO2-expanded DMF at 2.0 MPa (blue curves), 4.5 MPa (red curves) and 6.6 MPa (green curves). (b) The mesopore size distribution curves for the Cu3(BTC)2synthesized under the same conditions. Figure 3a shows the N 2 adsorption–desorption isotherms of the Cu 3 (BTC) 2 synthesized in CO 2 -expanded DMF at different pressures. They exhibit an intermediate mode between type I and type IV, which are related to mesoporous and microporous materials, respectively. The mesopore size distribution curves, calculated from Barrett–Joyner–Halenda analysis, are shown in Fig. 3b . The mesopore diameters of the Cu 3 (BTC) 2 synthesized at 2.0, 4.5 and 6.6 MPa are centred at 13, 20 and 23 nm, respectively. Evidently, higher CO 2 pressure favours the formation of larger mesopores, which is consistent with the scanning electron microscopic (SEM) observations. From N 2 adsorption–desorption isotherm, the diameter of the micropores was calculated to be 0.85 nm by Horvath–Kawazoe analysis ( Supplementary Fig. 6 ), in agreement with the micropore diameter estimated from crystallographic data of Cu 3 (BTC) 2 (ref. 37 ). The porosity properties of the MOFs were further characterized by small-angle X-ray scattering (SAXS) and the results are shown in Supplementary Fig. 7 . The SAXS profiles ( Supplementary Fig. 7A ) display power law scattering of Q −4 in the low Q region (Q<0.08 Å −1 ), corresponding to the asymptotic scattering behaviour of mesopores [43] . The mesopore size distributions of the MOFs synthesized at pressure of 2.0, 4.5 and 6.6 MPa were calculated, which are centred at about 13.8, 19.0 and 21.1 nm ( Supplementary Fig. 7B ). These results are consistent with the mesopore size distributions obtained from N 2 adsorption–desorption. The results prove the formation of hierarchically meso- and microporous MOFs in CXL and the mesopore size can be easily tuned by varying pressure. Figure 3: Porosity measurements. Porosity properties of Cu 3 (BTC) 2 determined by N 2 adsorption–desorption method. ( a ) N 2 adsorption–desorption isotherms of the Cu 3 (BTC) 2 synthesized in CO 2 -expanded DMF at 2.0 MPa (blue curves), 4.5 MPa (red curves) and 6.6 MPa (green curves). ( b ) The mesopore size distribution curves for the Cu 3 (BTC) 2 synthesized under the same conditions. Full size image The surface areas and pore volumes of the hierarchically porous Cu 3 (BTC) 2 synthesized in CO 2 -expanded DMF at different pressures are listed in Table 1 , as identified from the N 2 adsorption–desorption isotherms. The BET (Brunauer, Emmett and Teller) surface area ( S BET ) values of the three MOFs are not very high (~700 m 2 g −1 ), which can be ascribed to the pore impenetration [44] . The total pore volumes ( V t ) of the three MOFs are rather high (>1.28 cm 3 g −1 ). The micropore volume is around 0.2 cm 3 g −1 , while the mesopore volume ( V meso ) accounts for about 85% of the total pore volume of the MOFs. As far as we know, the MOFs synthesized in CO 2 -expanded DMF represent the largest mesopore volume value among the reported meso-MOFs (usually in the range of 0.1–0.5 cm 3 g −1 ). The ultra-high mesopore volumes of the as-synthesized Cu 3 (BTC) 2 result from their mesocellular structure. Moreover, Table 1 shows that the mesopore volume of the MOF synthesized in CO 2 -expanded DMF at higher pressure is larger, suggesting that more CO 2 dissolved in DMF is favourable to form mesopores in MOF. Materials with high pore volume as well as large mesopores would be of importance for their applications in diverse fields such as catalysis, drug delivery, separation and energy storage. Table 1 Porosity properties of the Cu 3 (BTC) 2 synthesized in CXLs. Full size table Mesoporous Cu 3 (BTC) 2 synthesized in other CXLs Furthermore, the Cu-BTC MOFs were synthesized in CO 2 -expanded N , N -dimethylacetamide (DMA) and N -methyl-2-pyrrolidone (NMP) at 4.5 MPa, respectively. They both have a large-pore mesoporous structure (see SEM images, XRD patterns and N 2 adsorption–desorption isotherms in Supplementary Figs 8–10 ), indicating that CO 2 is efficient for directing the assembly of mesocellular MOFs in different solvents. As listed in Table 1 , the porosity properties and the mesopore size are decreased in the order of DMF>DMA>NMP. To better understand the effect of CO 2 on the mesocellular MOF formation, the volume expansions (Δ V ) of the three organic solvents in CO 2 were determined. All these solvents can be expanded greatly by CO 2 , and the Δ V at the same pressure increases in the order of NMP<DMA<DMF ( Supplementary Fig. 11 ). By combining the results shown in Table 1 , evidently, the MOF synthesized in the more expanded liquid has higher porosity and larger mesopores. Formation mechanism On the basis of the experimental results, a possible mechanism for the CO 2 -directed formation of mesocellular MOF is proposed ( Fig. 4 ). First, the Cu 2+ ions react with the deprotonated BTC 3− to structure the nanosized framework building blocks [39] , [45] . Owing to the reduced solvency and viscosity of solvent by CO 2 expansion, the microporous MOF building blocks produced in the CO 2 -expanded solvent are expected to be smaller than those yielded in CO 2 -free solvent [39] , [45] , and higher pressure favours the formation of smaller building blocks [32] , [33] , [34] . In a second step, the nanosized MOF building blocks assemble to form the network because smaller particles have higher surface energy [46] , and the assembly of MOF nanocrystals is looser at higher pressure due to the greater expansion of the solvent. Therefore, after removing the solvent and releasing CO 2 , the mesocellular MOFs with large mesopores and thin mesopore walls are formed. The structural parameters of the MOFs are dependent on CO 2 pressure, that is, the higher the CO 2 pressure is, the more porous MOF with larger mesopores is formed. 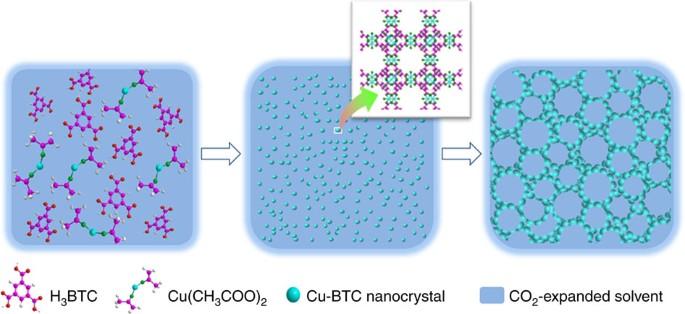Figure 4: Schematic illustration for mesocellular MOF formation. The Cu2+ions react with the deprotonated BTC3−in the CXL and the nanosized framework building blocks are produced. Then the MOF building blocks assemble to form the mesocellular MOFs with large mesopores and thin mesopore walls. Figure 4: Schematic illustration for mesocellular MOF formation. The Cu 2+ ions react with the deprotonated BTC 3− in the CXL and the nanosized framework building blocks are produced. Then the MOF building blocks assemble to form the mesocellular MOFs with large mesopores and thin mesopore walls. Full size image Catalytic activities of Cu 3 (BTC) 2 The Cu 3 (BTC) 2 MOFs synthesized in CO 2 -expanded DMF were used to catalyse the oxidation of benzyl alcohol to benzaldehyde, using 2,2,6,6-tetramethyl-piperidine-1-oxyl (TEMPO) as a co-catalyst [47] . The selectivity of benzaldehyde was >99%. As shown in Fig. 5a , the Cu 3 (BTC) 2 synthesized at higher pressure is more active. By using the Cu 3 (BTC) 2 synthesized at 6.6 MPa, benzyl alcohol converted completely to benzaldehyde at 3 h (red curve). The activities of the three MOFs are higher than that synthesized in pure DMF (black curve), further much higher than that of commercial Cu 3 (BTC) 2 at the same experimental conditions (10% conversion at 3 h) [47] . The catalyst shows no evident drop in catalytic activity after four runs ( Fig. 5b ), indicative of the high stability of the MOF. No notable difference was observed for the XRD patterns and SEM images of the fresh Cu 3 (BTC) 2 and that after being reused for four runs ( Supplementary Figs 12 and 13 ), indicating that the structural integrity of the MOF was well preserved. The porosity properties of the Cu 3 (BTC) 2 after being reused for four runs were determined by N 2 adsorption–desorption method ( Supplementary Fig. 14 ). The BET surface area of the recycled sample is 685 m 2 g −1 , which is slightly lower than that of the original sample (728 m 2 g −1 ). The mesopore size distribution of the recycled sample is nearly identical with that of the original one. This indicates that the mesoporous structure of the MOF can be well preserved after being reused for four runs. The slight drop of the BET surface area of the recycled MOF may be due to the presence of some inorganic and organic impurities generated during the reaction that blocks the micropore system [47] . 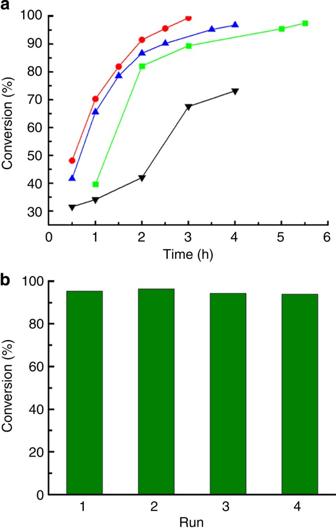Figure 5: Oxidation of benzyl alcohol using Cu3(BTC)2with oxygen. (a) Time conversion plot for the aerobic oxidation of benzyl alcohol to benzaldehyde catalyzed by the Cu3(BTC)2synthesized in CO2-expanded DMF at 2.0 MPa (green curve), 4.5 MPa (blue curve), 6.6 MPa (red curve) and in pure DMF (black curve). Reaction conditions: benzyl alcohol 0.185 mmol, catalyst 30 mg, DMF 1 ml, TEMPO (0.5 equiv), Na2CO3(1 equiv), 75 °C, oxygen atmosphere. (b) The reusability of the Cu3(BTC)2synthesized in CO2-expanded DMF at 6.6 MPa. Figure 5: Oxidation of benzyl alcohol using Cu 3 (BTC) 2 with oxygen. ( a ) Time conversion plot for the aerobic oxidation of benzyl alcohol to benzaldehyde catalyzed by the Cu 3 (BTC) 2 synthesized in CO 2 -expanded DMF at 2.0 MPa (green curve), 4.5 MPa (blue curve), 6.6 MPa (red curve) and in pure DMF (black curve). Reaction conditions: benzyl alcohol 0.185 mmol, catalyst 30 mg, DMF 1 ml, TEMPO (0.5 equiv), Na 2 CO 3 (1 equiv), 75 °C, oxygen atmosphere. ( b ) The reusability of the Cu 3 (BTC) 2 synthesized in CO 2 -expanded DMF at 6.6 MPa. Full size image Moreover, the catalytic activities of the as-synthesized mesoporous Cu 3 (BTC) 2 were tested for the aerobic oxidation of various alcohols. The reaction conditions are the same with those for the aerobic oxidation of benzyl alcohol. As can be known from Table 2 , 3-nitrobenzyl alcohol, 4-methylbenzyl alcohol and cinnamyl alcohol converted completely to the corresponding aldehydes in 10, 7 and 6 h, respectively (entries 1–3). By contrast, the aldehyde yields catalysed by the commercial microporous Cu 3 (BTC) 2 were 10, 65 and 62% for the three alcohols, respectively, even at a prolonged reaction time of 22 h (ref. 47 ). For the oxidation of 3,3′,5,5′-tetrakis(trifluoromethyl)benzhydrol catalysed by the mesoporous Cu 3 (BTC) 2 , the 3,3′,5,5′-tetrakis(trifluoromethyl)benzophenone yield reached 57.9% at 6 h, while that catalysed by the microporous Cu 3 (BTC) 2 was 18.7% at the same experimental conditions (entry 4). Such high catalytic activities of the Cu 3 (BTC) 2 synthesized in this work can be attributed to their mesocellular structure, which can enhance the diffusion of substrates and products [48] . Also, the nanoscale size of the MOFs is favourable for increasing the density of catalytic active sites [49] , thus accelerating the reaction more efficiently. Table 2 Oxidation of alcohols using Cu 3 (BTC) 2 with oxygen. Full size table Mesoporous Mn MOFs synthesized in CXL To expand the scope of the CXL for producing mesoporous MOF, we further performed the synthesis of other MOFs in the CXL. The mesoporous Mn-BTC and Mn-BDC (BDC=1,4-benzenedicarboxylate) MOFs were formed in the CO 2 -expanded DMF (see SEM images and XRD patterns in Supplementary Figs 15 and 16 ). The average mesopore size of the Mn MOFs is ~20 nm. The results indicate that the CXL is versatile in synthesizing different kinds of mesoporous MOFs. Here the mesocellular MOFs with large mesopores (13–23 nm) were synthesized in CXL. The porosity properties of the MOFs can be easily adjusted by controlling CO 2 pressure. The as-synthesized mesocellular Cu 3 (BTC) 2 MOFs are effective and reusable heterogeneous catalyst for the aerobic oxidation of benzylic alcohols under mild temperature at atmospheric pressure. By taking advantages of interconnected nature of the large mesopores, these mesocellular MOFs have potential applications in catalysis, gas separation and controlled drug release. The use of CXL for MOF formation has many advantages, for example, controllable, template-free and involves no longer ligand. It is worth noting that the Cu 3 (BTC) 2 MOF formation in organic solvent is usually carried out at temperature 70–180 °C and a reaction time longer than 10 h is needed [6] , [9] , [37] , [38] , [39] . Herein, the reaction in the presence of CO 2 proceeded at room temperature and the reaction time was shortened to 3 h. It can be attributed to the enhanced mass transport rates, resulting from the viscosity-lowering effect of CO 2 (ref. 22 ). Finally, we note that our method can be applied to the synthesis of different kinds of MOFs with large-pore mesoporous structure. Furthermore, we anticipate that the CXL could be used in the in situ production of mesoporous MOFs decorated with highly dispersed metal (or metal oxide) nanoparticles, which will find important applications in catalysis. Materials CO 2 (>99.95%) was provided by Beijing Analysis Instrument Factory. DMF and trifluoroacetate were provided by Beijing Chemical Reagent Company. DMA and NMP were purchased from J&K Scientific Co., Ltd. Cu(OAc) 2 ·H 2 O (A. R. Grade) was purchased from Alfa Aesar. H 3 BTC (purity 95%) was provided by Aldrich. Benzene dicarboxylic acid (H 2 BDC, 98%), MnCl 2 (97%), methyl ammonium (30 wt% H 2 O 2 ), benzyl alcohol (99%), cinnamyl alcohol (98%) and TEMPO (purity 98%) were supplied by Alfa Aesar. 3-Nitrobenzyl alcohol, 4-methylbenzyl alcohol and 3,3′,5,5′-tetrakis(trifluoromethyl)benzhydrol (purity 97%) were purchased from J&K Scientific Co., Ltd. Sodium carbonate was provided by Beijing Chemical Reagent Company. The methyl ammonium salt of the ligand H 2 BDC was made by dissolving the benzene dicarboxylic acid in a 40 wt % solution of methyl amine in water. The excess methyl amine and water were evaporated under reduced pressure, and the isolated salt was then redissolved in distilled water to give an aqueous solution of desired concentration. MOF synthesis In a typical experiment, H 3 BTC (0.25 mmol) and Cu(OAc) 2 ·H 2 O (0.5 mmol) were added into the solvent (5 g), which was loaded in a stainless steel autoclave (50 ml). Then 0.25 ml triethylamine was added into the autoclave to deprotonate the linker. CO 2 was charged into the cell under stirring until the desired pressure was reached. After the mixture was stirred at 30 °C for 3 h, the stirrer was stopped and the solvent was extracted by flowing CO 2 . The product was obtained after washing with ethanol for several times and drying at 60 °C under vacuum for 24 h. For comparison, the Cu-BTC MOF was synthesized in pure DMF, H 3 BTC (0.25 mmol) and Cu(OAc) 2 ·H 2 O (0.5 mmol) were added into DMF (5 g), which was loaded in a stainless steel autoclave (50 ml). Then 0.25 ml triethylamine was added into the autoclave to deprotonate the linker. After the mixture was stirred at 30 °C for 24 h, the stirrer was stopped. The product was obtained after centrifugation, washing with ethanol and drying at 60 °C under vacuum for 24 h. For the synthesis of Mn-BTC MOF, H 3 BTC (0.5 mmol) and MnCl 2 (0.5 mmol) were added into DMF (5 g), which was loaded in a stainless steel autoclave (50 ml). Then 0.25 ml triethylamine was added into the autoclave to deprotonate the linker. CO 2 was charged into the cell under stirring until the desired pressure was reached. After the mixture was stirred at 30 °C for 18 h, the stirrer was stopped. The product was obtained after washing with ethanol and drying at 60 °C under vacuum for 24 h. For the synthesis of Mn-BDC MOF, MnCl 2 (0.5 mmol) and the methyl ammonium salt of the ligand H 2 BDC (0.5 mmol) were added into DMF (5 g), which was loaded in a stainless steel autoclave (50 ml). The other experimental procedures and conditions were similar to those for the Mn-BTC MOF synthesis. MOF characterization The products were characterized by XRD (Model D/MAX2500, Rigaka) with Cu Kα radiation at a scanning rate of 5° min −1 . The morphologies were characterized by a HITACHI S-4800 scanning electron microscope. The porosity properties were gained from N 2 adsorption–desorption isotherms using a Micromeritics ASAP 2020M system. Fourier transform infrared spectra were obtained using a Bruker Tensor 27 spectrometer, and the samples were prepared by the KBr pellet method. The thermogravimetric measurements were carried out using Pyris 1 TGA with N 2 flow of 10 ml min −1 . The SAXS experiment was carried out at Beamline 4B9A at Beijing Synchrotron Radiation Facility. The wavelength was 1.38 Å and the distance of sample to detector was 2.044 m. Volume expansion The apparatus and experimental procedures were similar to those reported previously [50] . It consisted mainly of a high-pressure view cell of 50 ml, a constant temperature water bath, a high-pressure syringe pump (DB-80), a pressure gauge, a magnetic stirrer and a gas cylinder. The temperature of the water bath was controlled by a HAAKE D8 digital controller and the accuracy of the temperature measurement was ±0.05 K. The pressure gauge was composed of a pressure transducer (FOXBORO/ICT, Model 93) and an indicator, which was accurate up to ±0.025 MPa in the pressure range of 0–20 MPa. In a typical experiment, the desired amount of organic solvent was added into the cell, and the cell was placed in the constant temperature water bath (30 °C). After the thermal equilibrium had been reached, a suitable amount of CO 2 was charged into the high-pressure cell. The magnetic stirrer in the optical cell was started to accelerate the mixing of CO 2 and the liquid. The pressure was unchanged with time as equilibrium was reached. The volume of the solution at equilibrium condition was known from the level of the liquid surface, and the volume expansion coefficient could be calculated on the basis of the volumes of the liquid before and after dissolution of CO 2 . More CO 2 was charged and the volume of the liquid at another pressure was determined. Catalytic test The procedure of catalytic reaction was similar to those reported by Garcia and coworkers [47] . A 5 ml flask was charged with the required amount of catalyst, TEMPO, and sodium carbonate. To this mixture, 1 ml DMF was added followed by the appropriate quantity of alcohol. The mixture was stirred at 75 °C under oxygen atmosphere. After the desired time, the heterogeneous mixture was cooled and centrifuged. The liquid product was analysed by a gas chromatograph (Agilent 6820). For the reusability investigation, after 3 h of reaction the catalyst was recovered by centrifugation, washed with ethanol and dried under vacuum. Then the solid was reused for a consecutive run. How to cite this article: Peng, L. et al. Highly mesoporous metal–organic framework assembled in a switchable solvent. Nat. Commun. 5:4465 doi: 10.1038/ncomms5465 (2014).